Biomimetic virus-based colourimetric sensors Many materials in nature change colours in response to stimuli, making them attractive for use as sensor platform. However, both natural materials and their synthetic analogues lack selectivity towards specific chemicals, and introducing such selectivity remains a challenge. Here we report the self-assembly of genetically engineered viruses (M13 phage) into target-specific, colourimetric biosensors. The sensors are composed of phage-bundle nanostructures and exhibit viewing-angle independent colour, similar to collagen structures in turkey skin. On exposure to various volatile organic chemicals, the structures rapidly swell and undergo distinct colour changes. Furthermore, sensors composed of phage displaying trinitrotoluene (TNT)-binding peptide motifs identified from a phage display selectively distinguish TNT down to 300 p.p.b. over similarly structured chemicals. Our tunable, colourimetric sensors can be useful for the detection of a variety of harmful toxicants and pathogens to protect human health and national security. Many animals change their skin colours to communicate, to express mood, for camouflage, or to respond to environmental changes [1] , [2] , [3] . In the tissues of these animals, various nano and microscale components play roles in generating distinct colours and achieving rapid colour changes [4] , [5] . Inspired by nature, sensors are being developed that change colour in response to target chemicals by employing biomimetic structures and mechanisms. In particular, structurally coloured biomaterials, such as butterfly wings, beetle exocuticles, cephalopod skins, mammalian skins and avian skins/feathers [6] , [7] , [8] , [9] , [10] , [11] , [12] , [13] , [14] , provide insight into developing colourimetric sensors. These materials exhibit brilliant colours that are derived from their hierarchically organized structures and are resistant to photobleaching [7] . Furthermore, they can rapidly shift colours on exposure to chemical vapours due to structural and/or refractive index changes [15] . Therefore, both structurally coloured materials in nature and their synthetic analogues are being explored as simple and portable colourimetric sensor platforms [16] , [17] , [18] , [19] , [20] , [21] . A significant drawback of previous structural colour sensors is their limited intrinsic affinity for specific targets of interest (for example, explosives and pathogens) and resulting poor selectivity against analytes with similar chemical structures. Current methods to promote target specificity by either chemically incorporating specific recognition motifs or by synthesizing arrays of cross responsive platforms for ‘artificial nose’ type pattern recognition are promising [19] , [22] , [23] , [24] , but incorporating analyte-responsive elements into the sensing devices is still challenging because it requires complex designs and multistep synthetic pathways. Furthermore, many structurally coloured sensors exhibit viewing-angle dependent colour changes (iridescence) that may complicate analysis. Here we describe a bioinspired, colourimetric sensing material composed of filamentous bacterial viruses (M13 phage) as depicted in Fig. 1 . Tunable phage-based structures fabricated using a self-templating assembly process are composed of quasi-ordered phage-bundle nanostructures and exhibit viewing-angle independent colours [25] . These films mimic the structure of turkey skins ( Meleagris gallopavo , Pitman Farms, Sanger, CA, USA), which are structurally coloured blue due to coherent scattering of light from collagen bundle-based nanostructures ( Fig. 1a–c ) [11] . Arrays of differently coloured phage matrices, termed Phage litmus ( Fig. 1d ), rapidly swell or shrink on exposure to external chemicals, resulting in colour changes similar to those seen on turkeys when they get flustered ( Fig. 1a ). The chemicals are identifiable through colour pattern analyses in a quantitative manner. To enhance selectivity, a trinitrotoluene (TNT)-binding motif identified by phage display is incorporated onto the phage coats. The TNT-binding phage litmus detects TNT down to 300 p.p.b. with the aid of a common handheld device (iPhone) and can distinguish between similar nitroaromatic molecules (that is, TNT, dinitrotoluene (DNT) and mononitrotoluene (MNT)). The facile synthesis, ease of use, portability and successful introduction of tunable receptors suggest that Phage litmus colourimetric sensors can be useful for the detection of a wide variety of harmful toxicants and pathogens to protect human health and national security. 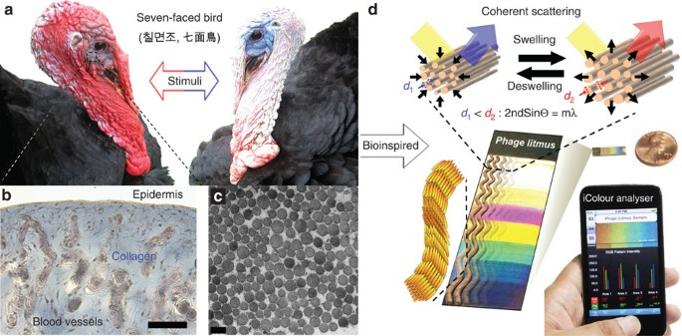Figure 1: Schematic of biomimetic colourimetric sensor system. (a) Turkeys autonomously change their red skin to white and/or blue when excited. The blue colour is associated with structural colourization of collagen nanostructures11, although their colour-change mechanism is not known with molecular detail. As a result, turkeys are known as ‘seven-faced birds’ in Korea and Japan. (b) A histological section of turkey skin stained with Masson’s trichrome shows that turkey skin consists mainly of collagen and highly vascularized tissues (scale bar, 50 μm). (c) Transmission electron micrograph of perpendicularly aligned collagen bundled fibres in the dermis (scale bar, 200 nm). (d) Bioinspired phage-based colourimetric sensors, termed Phage litmus, are composed of hierarchical bundles like the collagen fibres in turkey skins. Application of target molecules (chemical stimuli) causes colour shifts due to structural changes, such as bundle spacing (d1andd2) and coherent scattering. Using a handheld device’s camera (iPhone) and home-built software (iColour Analyser), we can identify target molecules in a selective and sensitive manner. Figure 1: Schematic of biomimetic colourimetric sensor system. ( a ) Turkeys autonomously change their red skin to white and/or blue when excited. The blue colour is associated with structural colourization of collagen nanostructures [11] , although their colour-change mechanism is not known with molecular detail. As a result, turkeys are known as ‘seven-faced birds’ in Korea and Japan. ( b ) A histological section of turkey skin stained with Masson’s trichrome shows that turkey skin consists mainly of collagen and highly vascularized tissues (scale bar, 50 μm). ( c ) Transmission electron micrograph of perpendicularly aligned collagen bundled fibres in the dermis (scale bar, 200 nm). ( d ) Bioinspired phage-based colourimetric sensors, termed Phage litmus, are composed of hierarchical bundles like the collagen fibres in turkey skins. Application of target molecules (chemical stimuli) causes colour shifts due to structural changes, such as bundle spacing ( d 1 and d 2 ) and coherent scattering. Using a handheld device’s camera (iPhone) and home-built software (iColour Analyser), we can identify target molecules in a selective and sensitive manner. Full size image Generation of multicolour Phage litmus We developed tunable, multicoloured, thin-film matrices composed of biomimetic fibre bundle nanostructures using M13 phage ( Fig. 2a ). M13 phage is a bacterial virus composed of single-stranded DNA encapsulated by 2,700 copies of the major coat protein (pVIII). Phages generate identical copies of themselves through infection of bacterial host cells. Because of its well-defined, monodisperse shape and its ability to display functional peptides, M13 phage has been utilized to fabricate various functional nanomaterials for semiconductor [26] , [27] , [28] , energy [29] , [30] , [31] and bioengineering applications [32] . Recently, inspired by self-templated materials assembly processes in nature, we developed a process to fabricate an array of hierarchical phage-based structures through controlled extraction of a solid substrate from a solution of phage ( Fig. 2b ) [25] . By controlling the phage deposition process, we could easily fabricate distinct and tunable structurally coloured nanostructures, in which colours do not appear to be strongly angle dependent. ( Fig. 2b , red box in Fig. 2c , Supplementary Figs 1 and 2 , and Supplementary Movie 1 ). Unlike typical synthetic photonic crystals that often rely on crystalline arrays or multilayer thin films [33] , [34] , the coloured regions of our self-templated materials were found to be composed of quasi-ordered fibre bundles that are remarkably similar to the collagen fibre bundles found in structurally coloured avian and mammalian skins [10] , [11] . Atomic force microscopy (AFM) and fast Fourier transform (FFT) analyses showed that the observed colours are attributable to coherent scattering from the fibre bundle structures ( Fig. 2b , Supplementary Figs 3 and 4 ). In quasi-ordered structures such as ours, the observed colours are determined by the average interparticle distance. A similar mechanism for angle-independent structural colour generation has been observed in animals and insects due to the presence of quasi-ordered dermal protein arrays [7] , [13] , [35] . 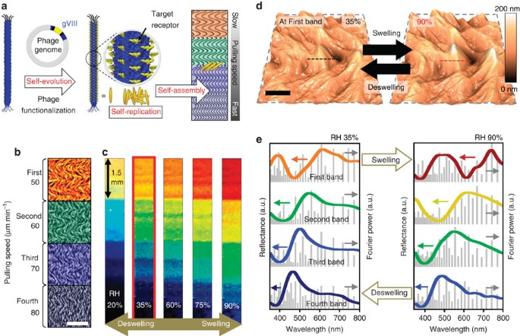Figure 2: Multicolour generation and structural modulation of the Phage litmus. (a) Phages genetically engineered to recognize target molecules through directed evolution, replicate to create identical copies and then self-assemble into coloured matrices composed of quasi-ordered bundled structures. (b) Composite of AFM images from different matrices (bands) of a Phage litmus. Each matrix is composed of quasi-ordered fibre bundles with different diameter and interspacing, and exhibits a different colour. (c) A fabricated Phage litmus exhibiting four distinct colours; orange, green, blue and deep blue (in red box). Changes in relative humidity (RH) result in changes in colours. Depending on the initial phage-bundle structure, each phage matrix swells with a different ratio and exhibits a different colour change. (d) AFM images of the first phage matrix band at 35% RH and 90% RH, respectively. Changes in colour are due to modulation of the phage bundles’ structures. Height profiles of the cross section (dotted lines) showed that bundle diameter increases 104 nm after swelling (Supplementary Fig. 6f). (e) Reflectance spectra (coloured lines) at normal angle and Fourier power spectra (grey bars) of each phage matrix in 35 and 90% RH generally correspond to each other in hue (position of peak) and chroma (shape of peak; a.u., arbitrary units). Figure 2: Multicolour generation and structural modulation of the Phage litmus. ( a ) Phages genetically engineered to recognize target molecules through directed evolution, replicate to create identical copies and then self-assemble into coloured matrices composed of quasi-ordered bundled structures. ( b ) Composite of AFM images from different matrices (bands) of a Phage litmus. Each matrix is composed of quasi-ordered fibre bundles with different diameter and interspacing, and exhibits a different colour. ( c ) A fabricated Phage litmus exhibiting four distinct colours; orange, green, blue and deep blue (in red box). Changes in relative humidity (RH) result in changes in colours. Depending on the initial phage-bundle structure, each phage matrix swells with a different ratio and exhibits a different colour change. ( d ) AFM images of the first phage matrix band at 35% RH and 90% RH, respectively. Changes in colour are due to modulation of the phage bundles’ structures. Height profiles of the cross section (dotted lines) showed that bundle diameter increases 104 nm after swelling ( Supplementary Fig. 6f ). ( e ) Reflectance spectra (coloured lines) at normal angle and Fourier power spectra (grey bars) of each phage matrix in 35 and 90% RH generally correspond to each other in hue (position of peak) and chroma (shape of peak; a.u., arbitrary units). Full size image Phage litmus-based humidity sensor The multicoloured Phage litmus exhibits structural responses on exposure to chemicals. The colour of each band of a Phage litmus red-shifted with increasing humidity and blue-shifted with decreasing humidity ( Fig. 2c ). Optical characterization showed that the reflectance spectra correlated to each visible colour ( Supplementary Fig. 5 ). When we increased the relative humidity from 35 to 90%, the observed wavelength of the reflectance spectrum increased ( Δλ =124 nm, 75 nm, 55 nm and 28 nm for the first, second, third and fourth band, respectively). AFM imaging analysis revealed that the changes in colour were due to modulation of the phage-bundle structures and subsequent thickness changes ( Fig. 2d ), with each band swelling to a different extent. When the relative humidity increased from 35% to 90%, the bundle diameter changed by 120 nm, 87 nm, 55 nm and 32 nm, and the band film thickness changed by 82 nm, 51 nm, 40 nm and 23 nm for the first, second, third and fourth matrices, respectively ( Supplementary Fig. 6 ). The most pronounced colour change was observed in the bands with the largest bundle diameters. FFT analyses of the AFM images also supported that the colour change was due to swelling and increased interspacing between fibre bundles ( Fig. 2e and Supplementary Fig. 4 ). During in situ grazing incidence small-angle X-ray scattering (GISAXS) experiments, the (100) and (110) peaks arising from the pseudohexagonally packed matrix structure gradually disappeared due to structural changes caused by the exposure to humidity ( Supplementary Fig. 7 ). Meanwhile, dynamic height measurements using AFM in a closed cell showed a structure change on exposure to water vapour within 20 s ( Supplementary Fig. 8 ). On removal of stimuli, the Phage litmus recovered its original colours within a few seconds ( Supplementary Fig. 9 ). The colour changes were observed repeatedly and reproducibly through more than a dozen cycles with little colour hysteresis ( Supplementary Movie 2 ). VOC detection using Phage litmus The Phage litmus exhibited characteristic colour changes when exposed to volatile organic compounds (VOCs). On exposure to hexane, diethyl ether, isopropyl alcohol, ethanol and methanol, the bands of the Phage litmus immediately changed colour. These changes were distinguishable to the naked eye at 300 p.p.m. of VOC ( Fig. 3a ). Quantitative real-time response to the organic solvents was recorded using a charge-coupled device (CCD) video camera controlled by a MATLAB programme for RGB (red, green and blue) colour component analysis ( Fig. 3b and Supplementary Fig. 10 ). Using this system, we found that the sensors exhibited distinct colour changes in response to the polarity index of the applied VOC ( Supplementary Figs 11 and 12 ). We then created a reference ‘fingerprint’ for each VOC by processing the amount the colours changed and generating synthetic colour patterns ( Fig. 3c and Supplementary Table 1 ). These references could be compared with the pattern generated by exposure to an unknown VOC to identify the sample’s identity. 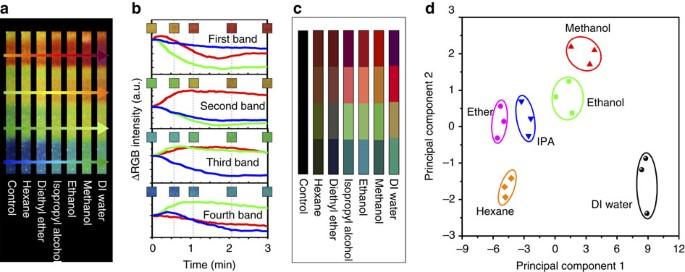Figure 3: Phage litmus sensing of gas phase VOCs. (a) Photographs of the Phage litmus after exposure to hexane, diethyl ether, isopropyl alcohol, ethanol, methanol and DI water, respectively. (b) Real-time RGB colour change profile of a Phage litmus after exposure to DI water. Each plot represents the RGB colour intensity change from each matrix of a Phage litmus. Time-dependent RGB colour change profiles for the other VOC-sensing experiments are shown inSupplementary Fig. 10. (c) VOC colour fingerprints used to selectively distinguish various chemicals. (d) Principal component analysis plot of the colour changes resulting from the exposure of the Phage litmus to different VOCs. Figure 3d shows a two-dimensional (2D) principal component analysis (PCA) plot containing points for each of the solvents from three measurements. The first two principal components account for 95% of the variance in the measurements. Clustering of data using PCA allows for assessment of the discrimination capabilities of the system and also demonstrates high reproducibility, as verified by the clustering of the data obtained for each solvent; deionized (DI) water (p1), methanol (p2), ethanol (p3), isopropyl alcohol (p4), diethyl ether (p5) and hexane (p6). On the basis of four different colourimetric matrices, we could clearly discriminate between the VOCs by polarity index; low-polarity VOCs tended to group together in the negative range of the plot, well separated from the high-polarity VOCs. Figure 3: Phage litmus sensing of gas phase VOCs. ( a ) Photographs of the Phage litmus after exposure to hexane, diethyl ether, isopropyl alcohol, ethanol, methanol and DI water, respectively. ( b ) Real-time RGB colour change profile of a Phage litmus after exposure to DI water. Each plot represents the RGB colour intensity change from each matrix of a Phage litmus. Time-dependent RGB colour change profiles for the other VOC-sensing experiments are shown in Supplementary Fig. 10 . ( c ) VOC colour fingerprints used to selectively distinguish various chemicals. ( d ) Principal component analysis plot of the colour changes resulting from the exposure of the Phage litmus to different VOCs. Full size image TNT detection using TNT–Phage litmus The M13 phage proved useful in detecting target materials with high selectivity and sensitivity, because target-specific phage can be identified through well-established phage display techniques [36] , [37] , [38] . We enhanced the selectivity of the Phage litmus by incorporating target-specific binding motifs identified through directed evolutionary screening of a combinatorial, phage-displayed peptide library. Although the Phage litmus composed of wild-type M13 phage gives a characteristic response for the various VOCs that have high vapour pressures, little colour change was observed in response to low-vapour-pressure organic compounds such as explosives or environmental toxicants. To demonstrate that such compounds could be specifically detected, we targeted TNT as a model explosive chemical. First, phages were engineered to display a TNT-binding peptide motif identified by phage display on their major coat proteins (DDWHWQEG; Fig. 4a ) [39] . After confirming the specific binding capability of the TNT-binding phage (TNT phage; Supplementary Fig. 13 ), we constructed TNT-phage-based colourimetric thin films (TNT–Phage litmus) and tested their TNT vapour-sensing capabilities. On exposure to TNT vapour, the TNT–Phage litmus exhibited sensitive and selective colour changes. As the concentration of applied TNT vapour increased, the TNT–Phage litmus showed pronounced colour changes due to structural changes induced by TNT binding ( Supplementary Fig. 14 ) and, as observed in the previous organic vapour experiments, the colour bands with wider diameter fibre bundles had more pronounced responses compared with those with narrower diameters. We believe that the colour changes resulted from structural modifications to the phage matrices induced by binding with the nitroaromatic target molecules. We confirmed TNT binding to TNT–Phage litmus through Fourier transform–infrared spectroscopy analyses ( Supplementary Fig. 15 ). When we exposed a Phage litmus composed of control phage displaying four glutamates (EEEE (4E)) to TNT, there were neither significant colour changes nor Fourier transform–infrared spectroscopy spectrum changes ( Supplementary Fig. 16 ). To enhance the accuracy and convenience of colourimetric analysis, we exploited the photographic and computational functions of common handheld devices (that is, iPhones). We utilized the device’s camera and a home-built analysis application, which we termed iColour Analyser, to produce 8-bit RGB colour components that can be used to easily quantify the colour change in each band of our sensors ( Supplementary Movie 3 ). Using the iColour Analyser, we could detect down to 300 p.p.b. of TNT in the gas phase ( Fig. 4b and Supplementary Fig. 17 ). We obtained a dissociation constant ( K d ) of 2.2 p.p.m. for the TNT–phage interaction with TNT ( Supplementary Fig. 18 ). To test the specificity of the phage matrices, we applied chemicals with similar structures to that of TNT (that is, DNT and MNT). On exposure to TNT (20 p.p.m. ), DNT (20 p.p.m.) and MNT (300 p.p.m.) vapour, the TNT–Phage litmus showed selective response to the TNT molecules, more than three and five times higher compared with DNT and MNT, respectively ( Fig. 4c and Supplementary Fig. 19 ). A 2D PCA plot supported the discrimination capabilities and reproducibility of the TNT–Phage litmus sensor ( Fig. 4d ). The first two principal components account for 97.2% of the variance in the three measurements of each chemical. Through the pattern recognition process, we could distinguish the target TNT, DNT and MNT down to 300 p.p.b. using our iColour Analyser system. We performed experiments in mixed vapours of ethanol, MNT, DNT and TNT to test the specificity of our TNT–Phage litmus sensor in the presence of interfering molecules. The TNT–Phage litmus showed negligible responses to relatively large amounts of MNT (20,000 p.p.m.) and DNT (400 p.p.m. ), while addition of 20 p.p.m. TNT vapour caused a significant colour change ( Supplementary Fig. 20a ). In a 300-p.p.m. ethanol background, the TNT–Phage litmus also responded selectively to TNT molecules ( Supplementary Fig. 20b ). This result demonstrates that our system selectively distinguishes TNT over other molecules with similar chemical structure in the presence of interferents. When our Phage litmus might exhibit a response to real-world interferents such as humidity or common VOCs, we can exclude nonspecific responses by comparison with the response of a non-sensitive Phage litmus. For example, the 4E–Phage litmus was non-responsive to TNT in the presence of ethanol, MNT and DNT ( Supplementary Fig. 20c ). 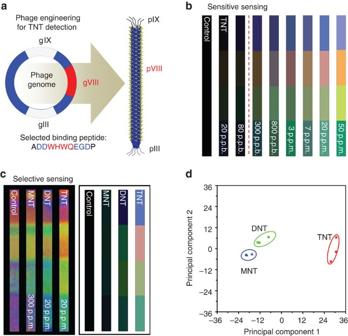Figure 4: Gas phase TNT detection using Phage litmus. (a) Two thousand and seven hundred copies of the TNT-binding receptor (WHWQ) identified by directed evolution are genetically engineered onto the surface of M13 phage (TNT phage). (b) Using the iPhone-based analysis system, TNT is detectable down to 300 p.p.b. in the gas phase. The dashed redline indicates the sensitivity limit of the TNT–Phage litmus against TNT. (c) Photos and processed colour fingerprints from the TNT–Phage litmus after TNT, DNT and MNT exposure. The TNT–Phage litmus selectively detects the target TNT (20 p.p.m.) over other molecules with similar chemical structures, such as DNT (20 p.p.m.) and MNT (300 p.p.m.). (d) PCA plot of the colour changes resulting from the exposure of the Phage litmus to TNT, DNT and MNT. Figure 4: Gas phase TNT detection using Phage litmus. ( a ) Two thousand and seven hundred copies of the TNT-binding receptor (WHWQ) identified by directed evolution are genetically engineered onto the surface of M13 phage (TNT phage). ( b ) Using the iPhone-based analysis system, TNT is detectable down to 300 p.p.b. in the gas phase. The dashed redline indicates the sensitivity limit of the TNT–Phage litmus against TNT. ( c ) Photos and processed colour fingerprints from the TNT–Phage litmus after TNT, DNT and MNT exposure. The TNT–Phage litmus selectively detects the target TNT (20 p.p.m.) over other molecules with similar chemical structures, such as DNT (20 p.p.m.) and MNT (300 p.p.m.). ( d ) PCA plot of the colour changes resulting from the exposure of the Phage litmus to TNT, DNT and MNT. Full size image We developed a facile, biomimetic, colourimetric sensing system to detect explosive molecules in a selective manner by exploiting the advantageous features of phage: their abilities to replicate, self-assemble and evolve. Our sensing matrices possess multiple advantages over conventional biosensors: first, we can easily fabricate multiple colourimetric matrices with tunable colours through a one-step self-assembly process. Importantly, these self-assembled matrices exhibit viewing-angle independent colours. Second, we can tailor the function of the phage matrices through directed evolution for specific target molecules and directly incorporate the target recognition motifs by genetic engineering. Furthermore, we can produce large-area multicolour matrices that are readable by a common handheld device. Our sensitive and selective colourimetric phage matrix sensors promise to establish rapid, portable and simple sensing. Although the TNT-sensing system was used as proof-of-concept in this study, this approach can be generalized to the detection of many harmful chemicals and biological toxicants. Genetic engineering of phage Our group identified a consensus TNT-binding peptide sequence (WHWQ) using phage display with a commercially available 12mer linear peptide library (Ph.D.-12) [37] , [39] . To incorporate the TNT-binding peptide, we genetically engineered the M13 phage’s major coat proteins (pVIII). The desired peptide sequences were inserted between the first and the sixth amino acids of the amino terminus of wild-type pVIII, replacing residues 2–5 (Ala- Glu-Gly-Asp-Asp -Pro to Ala-( Insert )-Pro) [32] . To incorporate the most stable phage to carry the consensus TNT-binding peptide (WHWQ) identified by phage display, we designed a partial library with sequence of the form A XX WHWQ XX DP using the primer: 5′-ATATATCTGCAG NKNNK TGGCATTGGCAG NNKN NKGAT CCCGCAAAAGCG GCCTTTAACTCCC-3′ and the primer 5′-GCTGTCTTTCGCTGC AGAGGGTG-3′ to linearize the vector ( N =A/C/G/T and K =G/T). To incorporate the gene sequences, PCR amplification was performed using Phusion DNA Polymerase, two primers (insertion and linearization) and an M13KE vector with an engineered Pst I site as the template. The obtained product was purified on an agarose gel, eluted by spin column purification, digested with Pst I enzyme and recircularized by an overnight ligation at 16 °C with T4 DNA ligase. The ligated DNA vector was transformed into XL1-Blue electroporation competent bacteria and the amplified plasmid sequence was verified at the University of California, Berkeley, DNA sequencing facility. The pVIII library was screened against TNT and the resulting sequences were tested for stability after large-scale amplification. The library member, ADDWHWQEGDP, was finally chosen to create our TNT–Phage litmus sensors. Alanine-substituted control phage (WAW, AHW and WHA) sequences were synthesized by site-directed mutagenesis of the WHW phage. Using similar genetic engineering approaches, we constructed 4E phage as a control. The constructed phages were amplified using bacterial cultures and purified through standard polyethylene glycol precipitation. The phage solution was further purified by filtration through 0.45 μm pore size membranes. To verify phage stability, DNA sequences were confirmed at each step of the amplification. Fabrication of Phage litmus We created the phage self-assembled colour band patterns using a simple pulling method [25] . The colours of the assembled structures were varied by controlling the pulling speed between 20 and 80 μm min −1 . We constructed a home-built phage deposition apparatus by modifying a syringe pump. We programmed software using C++ to control the motor speed (between 0.1 μm min −1 and 30 mm min −1 ) through an RS232C cable. For preparing Phage litmus matrices, we used 6 mg ml −1 4E phage suspensions in Tris-buffered saline (12.5 mM Tris and 37.5 mM NaCl, pH 7.5) or 2.4 mg ml −1 WHW-phage suspensions in DI water. A spectrum of coloured bands (each band was obtained at a different pulling speed) was clearly perceptible when the matrices were deposited on gold-coated Si wafers. Turkey skin sample preparation Fresh turkey head samples were donated from a local turkey farm (Pitman Farms, Sanger, CA, USA). The heads were obtained through overnight delivery immediately after they were slaughtered. The fresh turkey skin samples were immediately taken and processed for optical microscopy and transmission electron microscopy. For histology, ~0.5 × 1 cm turkey skin samples were soaked in 20% sucrose in PBS for 2 h, embedded in OCT Compound (Sakura, Torrance, CA, USA), cryosectioned at 5 μm thickness (Shandon Cryostat, Asheville, NC) and stained with Masson’s trichrome. Images were collected using an IX71 Microscope (Olympus, Tokyo, Japan). Transmission electron microscopy samples were fixed with 2% glutaraldehyde in 0.1 M sodium cacodylate (pH 7.2) for 1 h, post-fixed with 1% osmium tetroxide in 0.1 M sodium cacodylate (pH 7.2) and rinsed three times with sodium cacodylate (pH 7.2). Dehydration was done using a graded ethanol series (20, 40, 60, 80, 100 and 100%) followed by step-wise infiltration with epon-araldite resin (two parts acetone/one part resin for 1 h, one part acetone/one part resin for 1 h, one part acetone/two parts resin for 1 h, 100% resin for 1 h, 100% resin overnight, 100% resin with benzyl dimethylamine (BDMA) for 1 h) and heat polymerized in a 60 °C oven. Sample blocks were sectioned at 90 nm using a Leica EM UC6 microtome (Leica Microsystems Inc., Buffalo Grove, IL 60089, USA). Grids were stained with 2% uranyl acetate and Reynolds’ lead citrate. Imaging was done using a FEI Tecnai 12 transmission electron microscope (FEI, Hillsboro, OR 97124, USA). AFM analysis of Phage litmus AFM images were collected using an MFP3D AFM (Asylum Research, Santa Barbara, CA) and analysed using Igor Pro 6.0 (WaveMetrics, Inc., Lake Oswego, OR) and Asylum software package (Asylum Research). All images were taken in tapping mode with a tip spring constant of 2 N m −1 . The probe tips (Ted Pella, Inc., Redding, CA) were made of silicon with a 10-nm radius. The humidity experiments were carried out in a closed liquid cell. We injected a fixed quantity of DI water to control the humidity. FFT analysis of AFM cross-sectional height profiles was used to determine the periodicity of the self-assembled nanofilament structures within the Phage litmus matrices. Numerical computation of the Fourier transform was done with a 2D FFT algorithm in OriginPro 8 (Origin Lab Corp., Northampton, MA) and imageJ v1.44p (National Institutes of Health, USA). We calculated the Fourier power spectra expressed in spatial frequency (μm −1 ) from the AFM images. Reflectance measurements of Phage litmus Phage litmus matrices were illuminated by a white light source of a Xenon lamp (X-Cite, Exfo, Mississauga, Canada) and the reflected spectra were obtained using a fibre optic spectrophotometer (USB4000, Ocean Optics, Dunedin, FL) through a Y-shaped bifurcated optical fibre ( Supplementary Fig. 21 ). An optical fibre fixed on an x – y – z stage was positioned normal to the Phage litmus surface and perpendicular to the scanning direction. Reflectance was measured using a gold-coated Si wafer as a reference. The humidity experiments were performed in a closed glove box (Plas Labs, Inc., Lansing, MI). The humidity was controlled by DI water and monitored using a hygrometer (VWR International Inc., West Chester, PA). Reflectance measurements of Phage litmus under omnidirectional light To characterize the reflectance spectra of the Phage litmus under omnidirectional illumination, we lit a box coated with aluminium foil with a lamp (Incandescent Light, 150 W, DWC Sylvania, USA; Supplementary Fig. 22 ). We characterized the reflectance spectra while rotating the substrate between 10° and 90° from horizontal. A gold-coated Si wafer was used as a reference. Grazing incidence small-angle X-ray scattering To characterize the swelling behaviour of the Phage litmus, we performed in situ GISAXS experiments before and during exposure to humidity (~3 ml of DI water in a closed chamber). The GISAXS data were collected at the beamline 7.3.3 at the Advanced Light Source at Lawrence Berkeley National Laboratory. X-rays with a wavelength of 1.23984 Å (10 keV) were used, and the scattering spectra were collected on an ADSC Quantum 4 μm CCD detector with an active area of 188 × 188 mm (2,304 × 2,304 pixels). The scattering profiles were obtained after a 60-s collection time by integrating the 2D scattering pattern. The sample to detector distance was 1.84791, m and the incidence angle was 0.14°. Line-averaged intensities were reported as I versus q , where q =(4 π / λ ) × sin( θ /2), λ was the wavelength of incident X-rays and θ was the scattering angle. MATLAB-based analysis system for Phage litmus A home-built sensing and analysis system was developed for real-time chemical sensing. The equipment setup consisted of a gas chamber with an optical opening where a digital microscope (Celestron LLC, Torrance, CA) was attached to monitor the colour of the Phage litmus. The chamber with the Phage litmus inside was positioned on top of a heat block to control the temperature of the chamber. A MATLAB programme (Mathworks Inc., Natick, MA) was run on a PC to control the camera settings, to perform real-time readout and processing of the captured images and to display the real-time RGB data. First, the automatic gain of the digital microscope was turned to manual mode and a fixed gain was retained to prevent unwanted automatic compensation of brightness. The number of regions of interest, usually matching the number of different colour bands on the Phage litmus, was input by keyboard. Next, the specific regions to compare were selected from the first image (reference image) by mouse input. The subsequent images were taken and saved according to a pre-set frame rate (usually every 5 s). The change of the average RGB values with respect to the reference image for each region of interest was calculated and displayed on a graph in real time. We provide typical code from which we performed our experiments in Supplementary Note 1 . The vapour-phase experiments were performed by injection of a volume of solvent needed to achieve 300 p.p.m. concentration into a small container inside the chamber through an inlet tube. For explosive exposure experiments, we put excess amounts of each explosive crystal (200 mg) in a sealed chamber (20 ml) and controlled the vapour pressures by temperature. We obtained the concentration of all compounds based on the vapour pressure at each temperature with the assumption of vapour ideality. The vapour pressure of TNT, DNT and MNT was obtained from previously reported values [40] , [41] , [42] . To collect the data at saturated conditions, we held the Phage litmus in the sealed chamber for 30 min and then obtained corresponding sensing results. To test the specificity of our TNT–Phage litmus sensor towards interfering molecules, experiments were performed in mixed vapours of MNT, DNT and TNT. First, we put the small sealed chambers (1 ml) containing excess amounts of each explosive crystal (200 mg) in a large chamber with the phage litmus. Next, we exposed the chambers to MNT, DNT and TNT vapours sequentially using needles to open each small chamber ( Supplementary Fig. 20a ). A similar setup was used to perform the same experiments in a background of ethanol vapour ( Supplementary Fig. 20b ). We performed the control experiments using a 4E–Phage litmus sensor ( Supplementary Fig. 20c ). Surface plasmon resonance analysis Surface plasmon resonance analyses were performed using the Kretschmann optical configuration. A tungsten halogen lamp with a multiwavelength light source was used and a polarizer was positioned on the input path of the light for transverse magnetic fields. The prism coupler and the Phage litmus were mounted on an x–y–z stage. We made an enclosed cell of 100 μl using polydimethylsiloxane (PDMS) moulds. Flow of solution to the cell was implemented using 1 mm internal diameter tube. We injected 1 ml of solution into the cell at a flow rate of 50 μl min −1 . The outflow from the cell was carried through to a reservoir. The reflected spectrum was measured by a fibre optic spectrometer (USB4000-ultraviolet visible, Ocean Optics) and data acquisition was performed using a homemade LabVIEW programme (LabVIEW 2009, National Instrument, Austin, TX). The surface plasmon resonance spectrum was calculated from linearly polarized light parallel/perpendicular to the incidence plane (TM/TE configuration). iColour analyser iColour analyser is an iOS 5 application software built using the Xcode programming language (Xcode 4.2, Apple Inc., Cupertino, CA) and designed for the iPhone (Apple Inc, compatible with the iPod and iPad). This software has been built to analyse colourimetric changes of the RGB components from a Phage litmus in a systematic manner using a handheld device ( Supplementary Movie 3 ). As demonstrated in this paper, the RGB colour components and their changes from the Phage litmus can be linked to specific responses from target molecules. The iColour analyser workflow is constituted of different parts ( Supplementary Figs 23–26 ), as follows: Choice of analysis mode : A channel type (picker) is displayed to choose an analysis mode: single or double channel. Single-channel mode samples from one to five colour matrices of a Phage litmus labelled as S1–S5. The results display one to five different colour matrix RGB components in a bar graph and their values on an 8-bit level. Double-channel mode allows for colour comparison analysis between a reference Phage litmus (before exposure to chemical) and the sample Phage litmus (after exposure to chemical) through comparison between one and five matrices. The RGB values displayed will be the difference between the RGB values of the sample and the reference. Phage litmus sample (the picture sampler) : Once the user clicks on the single button of this application, the iPhone takes a picture of the Phage litmus. One can resize and crop the picture of the Phage litmus sample to precisely obtain the target area to analyse. Data analysis : Once the picture is taken, its central area is cropped and displayed. The picture is converted into a matrix containing the RGB and intensity values of each pixel. The vector data from the iPhone digital camera CCD (Omnivision OV5650, Santa Clara, CA) is processed to get the average of the RGB values from 2,592 × 1,944 pixels over the different areas selected by the user. An analysis table displays the RGB component intensity values and their s.d. An analysis graph will display the RGB values obtained from the sample. The ‘average’ picture displays a synthesized picture made from either the average RGB values in the case of the single analysis mode, or the difference between the average RGB values of the Phage litmus and its reference in the case of the double comparison mode. After displaying the analysis data and the date and time, a screenshot of the interface is saved in the picture browser of the iPhone and can be transferred easily to any computer through e-mail. In this work, for display purposes, the colour ranges of images are expanded from 5- to 8 bits per colour (RGB colour ranges of 0–31 expanded to 0–255). How to cite this article: Oh, J.-W. et al . Biomimetic virus-based colourimetric sensors. Nat. Commun. 5:3043 doi: 10.1038/ncomms4043 (2014).